An antioxidant nanozyme that uncovers the cytoprotective potential of vanadia nanowires Nanomaterials with enzyme-like properties has attracted significant interest, although limited information is available on their biological activities in cells. Here we show that V 2 O 5 nanowires (Vn) functionally mimic the antioxidant enzyme glutathione peroxidase by using cellular glutathione. Although bulk V 2 O 5 is known to be toxic to the cells, the property is altered when converted into a nanomaterial form. The Vn nanozymes readily internalize into mammalian cells of multiple origin (kidney, neuronal, prostate, cervical) and exhibit robust enzyme-like activity by scavenging the reactive oxygen species when challenged against intrinsic and extrinsic oxidative stress. The Vn nanozymes fully restore the redox balance without perturbing the cellular antioxidant defense, thus providing an important cytoprotection for biomolecules against harmful oxidative damage. Based on our findings, we envision that biocompatible Vn nanowires can provide future therapeutic potential to prevent ageing, cardiac disorders and several neurological conditions, including Parkinson’s and Alzheimer’s disease. Reactive oxygen species (ROS), such as superoxide, hydroxyl radicals and hydrogen peroxide, are generated as byproducts of cellular metabolism and from the Nox/Duox family of membrane-bound NADPH-dependent oxidases [1] , [2] . At lower concentrations, ROS serve as critical second messengers in various signalling pathways, whereas at higher concentrations, they exhibit detrimental effects [3] , [4] . Enhanced ROS levels are associated with oxidative damage to lipid, protein, DNA and activation of apoptotic pathways through induction of caspases [5] , [6] , [7] . It is also responsible for several pathological conditions such as neurodegeneration, cancer, diabetes, atherosclerosis, arthritis, kidney disorders and ageing [8] , [9] , [10] , [11] , [12] , [13] . Thus, regulation of ROS is crucial for the maintenance of cellular homeostasis. Cells produce several antioxidant enzymes, such as catalase, superoxide dismutase, glutathione peroxidase (GPx) and so on, to sustain the redox equilibrium [14] . Glutathione (GSH) acts as an electron donor to replenish the active form of enzyme and maintain cells’ reservoir of antioxidants [15] . The GSH-dependent GPx has a pancellular distribution with isoforms present in both cytosol and mitochondria, highlighting its significance in the maintenance of redox homeostasis [16] . Recently, organoselenium compounds having GPx-like antioxidant activity attracted considerable attention [17] , [18] . Nanomaterials with intrinsic enzyme-like activity attract significant current interest due to their ability to replace specific enzymes in enzyme-based applications [19] . A few nanostructured materials have been shown to mimic the activity of peroxidases [20] , [21] , oxidase [22] and superoxide dismutase [23] . Very recently, we reported the peroxynitrite isomerase and reductase activities of graphene–hemin hybrid nanosheets [24] . During our investigations on novel materials with interesting biological activities, we observed that V 2 O 5 , largely known as an oxidant [25] , [26] , can exhibit antioxidant activity at nanoscale. In this paper, we demonstrate that V 2 O 5 nanowires (Vn) exhibit remarkable antioxidant activity at physiologically relevant conditions. The internalization of Vn restores the ROS balance and controls the oxidative stress in the cell by catalytically reducing H 2 O 2 in the presence of GSH. Furthermore, Vn prevents oxidative damage to cellular components such as lipids, proteins and DNA, and thus plays a cytoprotective role in the cells. Synthesis and antioxidant activity Synthesis of Vn was carried out by a hydrothermal method as described earlier [27] . The nanomaterial was thoroughly characterized by various methods. Vn shows an absorption band at ~420 nm in the ultraviolet–visible spectrum ( Supplementary Fig. 1a ) corresponding to the bandgap of nano-V 2 O 5 , which is in agreement with the value reported earlier [28] . Scanning electron microscopy (SEM) and transmission electron microscopy (TEM) images indicate the nanowires of different sizes with width of ~100 nm and varying length ( Fig. 1a,b , respectively). High-resolution TEM image and selected area electron diffraction pattern confirm the formation of monocrystalline and orthorhombic V 2 O 5 ( Fig. 1c ). Electron dispersive X-ray (EDX) analysis shows the presence of V and O ( Supplementary Fig. 1b ). The formation of orthorhombic V 2 O 5 is also confirmed from the X-ray diffraction pattern (JCPDS # 001-0359) ( Fig. 1d ). 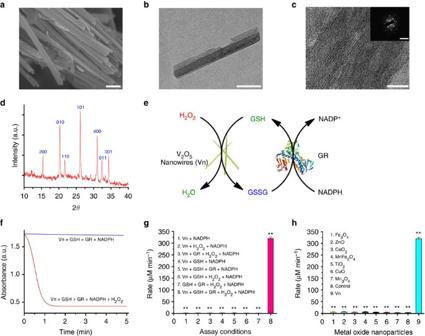Figure 1: Characterization and GPx-like activity of Vn. (a) SEM image of Vn showing the bunch of nanowires together. Scale bar, 200 nm. (b) TEM image of Vn. Scale bar, 100 nm (c) High-resolution TEM (HRTEM) image of Vn showing the planes and inset reveals the crystallinity and orthorhombic crystal structure of Vn. Scale bar, 10 nm (HRTEM), 10 nm−1(SAED). (d) Powder X-ray diffraction (XRD) of Vn where all the reflections are indexed to orthorhombic structure. (e) Schematic diagram depicting the GPx-like antioxidant activity of Vn and GSH recycling by GR. (f) Plot of absorbance versus time (min) revealing the activity of Vn in the presence of Vn (0.020 mg ml−1), GSH (2 mM), NADPH (0.4 mM), GR (1.7 units), H2O2(240 μM) in phosphate buffer (100 mM, pH 7.4) at 25 °C. When H2O2was absent in control, no reactivity was obtained. (g) Bar diagram showing the initial rates at different assay conditions. (h) Comparison of the GPx-like activity of various metal oxides that have been shown earlier as peroxidase and oxidase mimetics and Vn. Data represented as±s.e.m.,n=3, **P(t-test)<0.001. Figure 1: Characterization and GPx-like activity of Vn. ( a ) SEM image of Vn showing the bunch of nanowires together. Scale bar, 200 nm. ( b ) TEM image of Vn. Scale bar, 100 nm ( c ) High-resolution TEM (HRTEM) image of Vn showing the planes and inset reveals the crystallinity and orthorhombic crystal structure of Vn. Scale bar, 10 nm (HRTEM), 10 nm −1 (SAED). ( d ) Powder X-ray diffraction (XRD) of Vn where all the reflections are indexed to orthorhombic structure. ( e ) Schematic diagram depicting the GPx-like antioxidant activity of Vn and GSH recycling by GR. ( f ) Plot of absorbance versus time (min) revealing the activity of Vn in the presence of Vn (0.020 mg ml −1 ), GSH (2 mM), NADPH (0.4 mM), GR (1.7 units), H 2 O 2 (240 μM) in phosphate buffer (100 mM, pH 7.4) at 25 °C. When H 2 O 2 was absent in control, no reactivity was obtained. ( g ) Bar diagram showing the initial rates at different assay conditions. ( h ) Comparison of the GPx-like activity of various metal oxides that have been shown earlier as peroxidase and oxidase mimetics and Vn. Data represented as±s.e.m., n =3, ** P ( t -test)<0.001. Full size image To study the antioxidant activity of the water dispersible Vn, the glutathione reductase (GR) coupled assay was employed and the decrease of NADPH concentration was monitored spectrophotometrically at 340 nm [29] . Figure 1e shows the schematic representation of the GPx-like activity of Vn. In the absence of at least one of the components in the reaction mixture, Vn did not show GPx activity ( Fig. 1f,g and Supplementary Fig. 2a ). Although the reduction of vanadate (V) by GR in the presence of NADPH has been shown to represent a new pathway for vanadate metabolism [30] , such reduction by GR was not observed for Vn. The initial rates determined for the reactions of Vn with GR and H 2 O 2 in the presence of NADPH were very similar to that of the control reactions without H 2 O 2 ( Supplementary Fig. 2c,d ). Interestingly, none of the peroxidase or oxidase nanozymes reported earlier exhibit the unique activity of Vn under similar reaction conditions ( Fig. 1h ). The reactivity of Vn appears to be different from that of the other peroxidase nano-mimetics, where ·OH mediates the oxidation of organic substrates in the presence of metal ions. The remarkable selectivity of Vn towards H 2 O 2 is probably due to the activation of H 2 O 2 by Vn to produce a polar peroxido species instead of OH radical [27] , [31] . The peroxido species reacts further with the nucleophile (GSH cofactor) to form glutathione disulfide (GSSG) ( vide infra ). The supernatant liquid obtained after incubation of Vn for 15 min in the assay buffer did not show any noticeable antioxidant activity, indicating that the reaction occurs on the surface of Vn ( Supplementary Fig. 2b ). When the concentration of Vn was varied from 0 to 0.02 mg ml −1 in the presence of other required reagents, a proportional dependence of initial rate was observed for the reduction of H 2 O 2 ( Fig. 2a ) with first-order reaction kinetics ( Fig. 2a , inset). The apparent steady-state kinetic parameters were determined by independently varying the concentrations of H 2 O 2 (0–480 μM) and GSH (0–6.0 mM) in the presence of GR (1.7 units) and NADPH (400 μM). A typical Michaelis–Menten kinetics was observed for both the reactions ( Fig. 2b,c ). The Michaelis constant K M values, obtained from the corresponding Lineweaver–Burk plots ( Supplementary Fig. 3a,b ), for H 2 O 2 and GSH are ~0.11 and ~2.22 mM, respectively. These values are different from those obtained for GPx1 enzyme isoform ( K M for H 2 O 2 ~0.025 mM and GSH ~10 mM) [32] , [33] , indicating different binding affinity for the substrates. Vn catalyses the reaction at the maximal reaction velocity V max of ~0.43 and 0.83 mM min −1 for H 2 O 2 and GSH, respectively, with k cat =0.065 s −1 . Although GSSG is produced in the overall reaction, the Michaelis–Menten and Lineweaver–Burk profiles indicate that one GSH molecule is involved in the rate-determining step ( Supplementary Fig. 3c–e ). 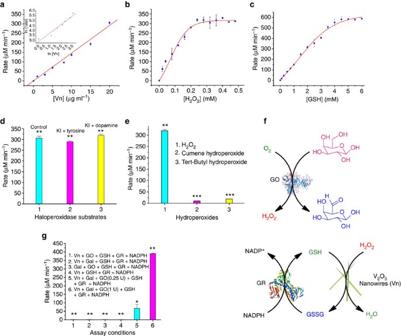Figure 2: Kinetic parameters and cooperativity studies. (a) Effect of concentration of Vn on the GPx-like activity showing the first-order kinetics as found in the enzyme catalysed reactions. Inset represents the plot of ln (rate) versus concentration of Vn. (b) Michaelis–Menten plot for the variation of the concentration of H2O2(0–0.48 mM) and in the presence of Vn ( 0.020 mg ml−1), GSH (2 mM), NADPH (0.4 mM), GR (1.7 units) in phosphate buffer (100 mM, pH 7.4) at 25 °C. (c) Michaelis–Menten plot for the variation of the concentration of GSH (0–6.0 mM) and in the presence of Vn (0.020 mg ml−1), NADPH (0.4 mM), GR (1.7 units), H2O2(240 μM) in phosphate buffer (100 mM, pH 7.4) at 25 °C. (d) Effect of the haloperoxidase substrate KI (2 mM), tyrosine or dopamine (2 mM) on the GPx-activity of Vn, showing that Vn preferably exhibits GPx-like activity and not haloperoxidase activity at pH 7.4. (e) Comparison of the reactivity of three different peroxides, H2O2,t-BuOOH and Cum-OOH. It shows that Vn is very selective to H2O2as substrate. (f) Schematic diagram of coupling GO with Vn nanozyme. The H2O2producedin situby GO was directly used by Vn for its GPx activity. This proves that the Vn shows cooperativity with other enzymes. (g) Bar diagram showing the initial rates, which are directly related to the cooperativity of Vn with different concentrations of GO (0.25 and 1 unit). The reaction occurs only when all the components are present. Data represented as±s.e.m.,n=3, **P(t-test)<0.001. Figure 2: Kinetic parameters and cooperativity studies. ( a ) Effect of concentration of Vn on the GPx-like activity showing the first-order kinetics as found in the enzyme catalysed reactions. Inset represents the plot of ln (rate) versus concentration of Vn. ( b ) Michaelis–Menten plot for the variation of the concentration of H 2 O 2 (0–0.48 mM) and in the presence of Vn ( 0.020 mg ml −1 ), GSH (2 mM), NADPH (0.4 mM), GR (1.7 units) in phosphate buffer (100 mM, pH 7.4) at 25 °C. ( c ) Michaelis–Menten plot for the variation of the concentration of GSH (0–6.0 mM) and in the presence of Vn (0.020 mg ml −1 ), NADPH (0.4 mM), GR (1.7 units), H 2 O 2 (240 μM) in phosphate buffer (100 mM, pH 7.4) at 25 °C. ( d ) Effect of the haloperoxidase substrate KI (2 mM), tyrosine or dopamine (2 mM) on the GPx-activity of Vn, showing that Vn preferably exhibits GPx-like activity and not haloperoxidase activity at pH 7.4. ( e ) Comparison of the reactivity of three different peroxides, H 2 O 2 , t -BuOOH and Cum-OOH. It shows that Vn is very selective to H 2 O 2 as substrate. ( f ) Schematic diagram of coupling GO with Vn nanozyme. The H 2 O 2 produced in situ by GO was directly used by Vn for its GPx activity. This proves that the Vn shows cooperativity with other enzymes. ( g ) Bar diagram showing the initial rates, which are directly related to the cooperativity of Vn with different concentrations of GO (0.25 and 1 unit). The reaction occurs only when all the components are present. Data represented as±s.e.m., n =3, ** P ( t -test)<0.001. Full size image As V 2 O 5 nanoparticles generally exhibit vanadium haloperoxidase mimetic activity [27] , we monitored the reaction of Vn with H 2 O 2 in the presence of vanadium haloperoxidase substrates, that is, tyrosine/iodide or dopamine/iodide. However, the rate of the reactions was unaffected ( Fig. 2d ) on introduction of the haloperoxidase substrates into the reaction mixture. This is probably due to the greater nucleophilic character of GS − over halide, which helps in a facile attack of GS − at the polarized oxygen atoms of the vanadium peroxido species formed on the surface of Vn on reaction with H 2 O 2 . The observed difference can also be attributed to the differential binding affinity of the two substrates for the catalyst. A comparison of the reaction rates for various peroxides H 2 O 2 , t -butyl hydroperoxide and cumene hydroperoxide indicates that the antioxidant activity of Vn is specific to H 2 O 2 ( Fig. 2e ). Although nanozymes are known to have incompatibility with a cascade of other enzymes [19] , we found that Vn has an excellent compatibility with galactose oxidase (GO) and GR in series ( Fig. 2f,g ). As GO can work efficiently with Vn, the decrease in the concentration of NADPH during the catalysis directly correlates with the galactose levels. Therefore, Vn can be used for sensing galactose when coupled with GO and GR. It is known that the quantitative measurement of galactose is important in food industry and in medical monitoring and treatment of patients. To understand the reactivity of Vn towards other biologically relevant oxidants, such as peroxynitrite (ONOO − , PN), we carried out the PN-mediated nitration of L -tyrosine and bovine serum albumin in the presence and absence of Vn. Although GSH and small molecule GPx mimetics such as ebselen have been shown to scavenge PN efficiently [17] , [18] , Vn does not react with PN as the nitration reactions were not affected by different concentrations of Vn ( Supplementary Fig. 4 ). Internalization of Vn in mammalian cells To understand the antioxidant activity of Vn nanozyme in cellular environment, we carried out cell-based studies. The cellular uptake of Vn was studied through three different approaches. First, the internalization of Vn in HEK293T (human embryonic kidney) cells was observed by SEM. Vn-treated cells showed the formation of depressions on the surface, which was absent in the untreated controls. However, the cells recovered after 2 h post treatment showed diminished indentation and restoration of surface morphology. This shows that the uptake of Vn probably occurs through endocytosis ( Fig. 3a,b and Supplementary Fig. 5 ). To further ascertain that the endocytotic depressions were due to uptake of Vn, we carried out an EDX analysis on the concavity. The specific peak corresponding to the vanadium was observed in the Vn-treated cells ( Fig. 3c,d ). Second, the internalization and presence of Vn were verified by observing the alterations in scattering pattern of a laser beam by the intracellular nanowires [34] , [35] . The concomitant increase in the Vn concentration caused a comparable variation in the scatter pattern, indicating an enhanced intracellular presence of Vn ( Fig. 3f,g ). Lastly, we assessed quantitatively the percentage uptake of Vn in the cells by inductively coupled plasma atomic emission spectroscopy (ICP-AES) by analysing the amount of vanadium in the cells. In comparison with the untreated control, we found a significant increase of vanadium levels in the treated cells, which corresponds to ~2.5% of the total Vn added to the cell population ( Fig. 3h ). These observations indicate that Vn is efficiently internalized into the cell albeit in lower amounts, probably through endocytotic mechanism. 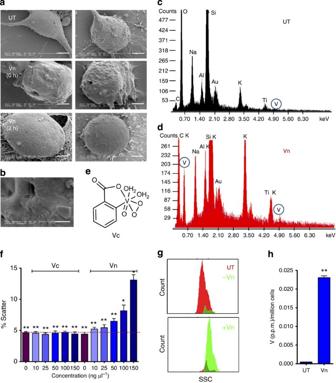Figure 3: Internalization of Vn in the cell. (a,b) HEK293T (human embryonic kidney) cells were either left untreated (UT), treated with Vn and immediately harvested (0 h) or recovered for 2 h post Vn exposure, before fixation, dehydration and imaging by scanning electron microscope;brepresents the zoomed image of the middle panel to highlight the depression. Scale bars, 2 μm (a) and 500 nm (b). (c,d) The cell surface depressions resulting due to Vn internalization was verified by EDX analysis on the depressed regions. Representative EDX plots depicting the absence and presence of vanadium peak in untreated (UT) and Vn-treated cells, respectively. (e) Structure of Peroxido vanadium picolinate complex (Vc). (f,g) The presence of Vn in the cells were assessed by flow cytometric analysis of altered side scatter intensity (SSC) resulting due to differential density of the intracellular Vn accumulation. HEK293T cells were treated with increasing concentrations of Vn and subjected to flow cytometric analysis. Soluble Vc-treated cells were used as negative controls. (g) Representative SSC histograms of cells kept either untreated (UT) or treated with 100 ng μl−1Vn. Data represented as mean±s.e.m.n=3, **P(t-test)<0.001, *P(t-test) <0.01. (h) The relative uptake of Vn by the cells was measured by ICP-AES and represented as amount of vanadium uptake per million cells with respect to untreated controls. Figure 3: Internalization of Vn in the cell. ( a , b ) HEK293T (human embryonic kidney) cells were either left untreated (UT), treated with Vn and immediately harvested (0 h) or recovered for 2 h post Vn exposure, before fixation, dehydration and imaging by scanning electron microscope; b represents the zoomed image of the middle panel to highlight the depression. Scale bars, 2 μm ( a ) and 500 nm ( b ). ( c , d ) The cell surface depressions resulting due to Vn internalization was verified by EDX analysis on the depressed regions. Representative EDX plots depicting the absence and presence of vanadium peak in untreated (UT) and Vn-treated cells, respectively. ( e ) Structure of Peroxido vanadium picolinate complex (Vc). ( f , g ) The presence of Vn in the cells were assessed by flow cytometric analysis of altered side scatter intensity (SSC) resulting due to differential density of the intracellular Vn accumulation. HEK293T cells were treated with increasing concentrations of Vn and subjected to flow cytometric analysis. Soluble Vc-treated cells were used as negative controls. ( g ) Representative SSC histograms of cells kept either untreated (UT) or treated with 100 ng μl −1 Vn. Data represented as mean±s.e.m. n =3, ** P ( t -test)<0.001, * P ( t -test) <0.01. ( h ) The relative uptake of Vn by the cells was measured by ICP-AES and represented as amount of vanadium uptake per million cells with respect to untreated controls. Full size image Intracellular ROS scavenging activity of Vn To test the ability of Vn to combat oxidative stress in the cells, we used two different approaches. The HEK293T cells pretreated with the nanoparticles were either treated exogenously by H 2 O 2 or the intrinsic cellular levels of peroxides were elevated by inhibiting the antioxidant enzyme catalase using either Cu 2+ ions [36] or 3-amino,1,2,4 triazole (3-AT) [37] . For the selection of appropriate concentrations of H 2 O 2 and Vn, the cells were treated with increasing concentration of H 2 O 2 and Vn for 15 min followed by measurement of cell viability and levels of cellular ROS using dihydrodichloro-fluoresceindiacetate (DCFDA-H2) probe ( Supplementary Fig. 6b–d ). Based on the relative fluorescence and cellular viability observed, 200 μM H 2 O 2 and 50 ng μl −1 of Vn were used for further experiments. Inhibiting the intracellular catalase in the presence of Vn highlights the ability of Vn to act as GPx enzyme mimetic by restoring the redox state and viability of the cells. To measure the scavenging of H 2 O 2 by Vn under stress conditions, we expressed a genetically encoded H 2 O 2 -specific probe HyPer and analysed the intracellular peroxide levels. The level of H 2 O 2 was found to decrease in the cells pretreated with Vn, whereas the cells treated either with only H 2 O 2 or Cu 2+ , or 3-AT showed enhanced levels of H 2 O 2 ( Fig. 4a,c ). Similarly, staining the cells with H 2 O 2 -specific dye Amplex Red and ROS-sensitive fluorescent dye DCFDA-H2 resulted in the detection of relatively lower ROS levels in Vn-pretreated cells under normal and oxidative stress conditions as compared with that of controls. Consistently, a substantial increase in the ROS levels was observed in the cells treated with either H 2 O 2 or Cu 2+ , or 3-AT alone as measured by flow cytometric analysis ( Fig. 4b,d and Supplementary Fig. 7a,b ). To test the utilization of GSH as a cofactor by Vn, the intracellular GSH was depleted by allyl alcohol (AA) [38] or buthionine sulfoximine (BSO) [39] , which resulted in loss of antioxidant function and an increase in the ROS. The antioxidant function was, however, restored on exogenous addition of GSH ( Fig. 4a–d and Supplementary Fig. 7a,b ). The broader effect of Vn was analysed using cells of diverse origin such as HeLa cells (cervical cancer), LNCaP (prostate cancer) and SH-SY5Y cells (neuroblastoma). In congruence to HEK293T cells, Vn showed similar H 2 O 2 scavenging ability in other cells as observed through microscopic analysis and flow cytometry ( Fig. 4e,f and Supplementary Fig. 8 ). This indicates that Vn nanozyme possesses intracellular ROS scavenging activity and its antioxidant function is mediated by GPx-like activity. In contrast, treatment of the cells with peroxido-vanadium-picolinate complex (Vc) ( Fig. 3e ), other similar complexes Vc 2 and Vc 3 ( Supplementary Fig. 7i ), and different forms of V 2 O 5 such as bulk-V 2 O 5 (Vb) and V 2 O 5 -foam (Vf) caused an increment in the cellular peroxides, which were further elevated on additional H 2 O 2 or Cu 2+ treatment ( Supplementary Fig. 7f ). These observations are in agreement with the fact that vanadium complexes can undergo redox reaction and generate ROS in cells [40] , [41] , [42] . Although V 2 O 5 is known to cause severe oxidative stress in cells [25] , [26] , in nano-form, it shows remarkable antioxidant GPx activity. It should be noted that complex Vc undergoes redox reactions without changing the ligand environment. Complex Vc exhibited a signal at −598 p.p.m. in the 51 V NMR spectrum, which disappeared completely on treatment with GSH. The product is a V(IV) complex and, hence, electron paramagnetic resonance active. However, when the reaction mixture was treated with H 2 O 2 , the signal at −598 p.p.m. reappeared ( Supplementary Fig. 6e ). 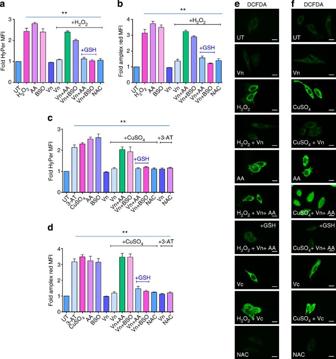Figure 4: Ability of Vn to scavenge intracellular ROS. (a,b) H2O2scavenging activity of Vn was measured using genetically encoded H2O2-specific probe HyPer in HEK293T cells. Cells were either left untreated or pretreated with 50 ng μl−1of nano-V2O5(Vn) prior exposure to 200 μM H2O2or 500 μM CuSO4, or 20 mM 3-amino-1,2,4-triazole (3-AT). AA (0.1 mM) or 50 μM BSO was used to deplete cellular GSH level. GSH (100 μM) was used to replenish the GSH level to show the requirement of GSH as a cofactor for Vn. To measure the ROS scavenging ability of vanadium complex (Vc), 50 ng μl−1Vc was used to treat the cells in the presence or absence of oxidative stress. N-acetyl cysteine-treated cells (NAC) (100 μM) were used as positive control. Data represented as mean±s.e.m.n=3, **P(t-test) <0.001. (c,d) To further confirm, the H2O2scavenging ability of Vn, HEK293T cells were subjected to various treatments as mentioned earlier and stained with H2O2-specific dye Amplex Red (50 μM). The fluorescence was measured at 590 nm using spectrofluorometer and data were represented as fold change in mean fluorescent intensity (MFI) of Amplex Red over untreated cells. Data represented as mean±s.e.m.n=3, **P(t-test)<0.001. (e,f) HeLa cells were treated with Vn before the treatment with H2O2(e) or CuSO4(f) (as mentioned earlier) and then stained with 15 μM DCFDA-H2 dye. The change in fluorescent intensity was observed through microscopic analysis (scale bar, 10 μm). Figure 4: Ability of Vn to scavenge intracellular ROS. ( a , b ) H 2 O 2 scavenging activity of Vn was measured using genetically encoded H 2 O 2 -specific probe HyPer in HEK293T cells. Cells were either left untreated or pretreated with 50 ng μl −1 of nano-V 2 O 5 (Vn) prior exposure to 200 μM H 2 O 2 or 500 μM CuSO 4 , or 20 mM 3-amino-1,2,4-triazole (3-AT). AA (0.1 mM) or 50 μM BSO was used to deplete cellular GSH level. GSH (100 μM) was used to replenish the GSH level to show the requirement of GSH as a cofactor for Vn. To measure the ROS scavenging ability of vanadium complex (Vc), 50 ng μl −1 Vc was used to treat the cells in the presence or absence of oxidative stress. N-acetyl cysteine-treated cells (NAC) (100 μM) were used as positive control. Data represented as mean±s.e.m. n =3, ** P ( t -test) <0.001. ( c , d ) To further confirm, the H 2 O 2 scavenging ability of Vn, HEK293T cells were subjected to various treatments as mentioned earlier and stained with H 2 O 2 -specific dye Amplex Red (50 μM). The fluorescence was measured at 590 nm using spectrofluorometer and data were represented as fold change in mean fluorescent intensity (MFI) of Amplex Red over untreated cells. Data represented as mean±s.e.m. n =3, ** P ( t -test)<0.001. ( e , f ) HeLa cells were treated with Vn before the treatment with H 2 O 2 ( e ) or CuSO 4 ( f ) (as mentioned earlier) and then stained with 15 μM DCFDA-H2 dye. The change in fluorescent intensity was observed through microscopic analysis (scale bar, 10 μm). Full size image The adaptability of the cells to nanowire treatment, the cytotoxicity of Vn and its ability to suppress ROS-induced apoptosis was analysed by MTT (3-(4,5-dimethylthiazol-2-yl)-2,5-diphenyltetrazolium bromide) assay, caspase 3/7 activation and propidium iodide staining. Treatment of cells with Vn alone did not alter the overall viability of the cells as compared with controls. However, it had a significant cell protective role and inhibited apoptosis under H 2 O 2 or Cu 2+ or 3-AT treatment. Consistent to the loss of antioxidant properties of Vn on GSH depletion, AA and BSO caused a decrease in the cell viability, which was reverted on addition of exogenous GSH ( Fig. 5a–d and Supplementary Fig. 7c,d ). This supports the idea that Vn possesses a GPx-like activity and uses GSH as a co-factor. To further confirm the cofactor requirement for the catalysis, the cellular GSH and GSSG levels were measured after treatment with Vn. Although no significant changes in GSH and GSSG levels were observed in the presence of Vn alone, an increase in the GSSG level (by ~1.5-fold) and a slight decrease in the GSH level (by~0.8-fold) was observed when the cells pretreated with Vn were exposed to H 2 O 2 ( Fig. 5e,f and Supplementary Fig. 9a ). Although two molecules of GSH are oxidized to form one GSSG molecule, the observed increase in the GSSG level did not result in a significant reduction in GSH level. This confirms that Vn uses GSH as a cofactor to scavenge H 2 O 2 , without compromising the recycling of GSSG to GSH. 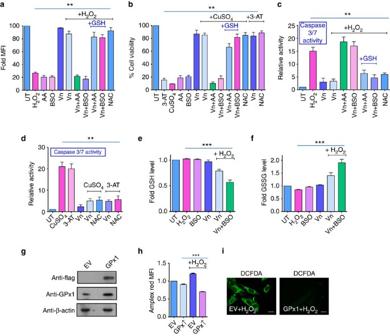Figure 5: Rescue of cell viability by Vn. (a,b) The viability of HEK293T cells under H2O2- or CuSO4-treated conditions along with other ROS modulators was observed through MTT assay and represented as mean±s.e.m.;n=8, **P(t-test)<0.001. (c,d) Prevention of ROS-mediated apoptosis induction by nano-V2O5was analysed through the effector caspase-3/7 activity by measuring cleavage of specific substrate, resulting in the increase in fluorescence intensity. Bars denote the fold intensity over untreated cells as mean±s.e.m.;n=3, ***P(t-test) <0.0001. (e,f) The level of cellular GSH or GSSG was quantified in HEK293T cells treated with Vn and GSH inhibitor (BSO) using GSH/GSSG-Glo kit (Promega). Data are represented as mean±s.e.m.;n=3, ***P(t-test) <0.0001. (g–i) The GPx mimetic nature of Vn was confirmed by overexpressing GPx1 in HEK293T cells. Cells were transfected with pCDNA3.1a empty vector (EV) or vector containing GPx1. GPx1 overexpression was analysed in whole-cell lysate using the anti-GPx1 antibody (g). Anti-Flag tag antibody and anti-β-actin antibodies were used as transfection control and loading control, respectively. The cellular H2O2level was measured by staining the cells with Amplex Red after 48 h of transfection (h). Results are presented as fold change in MFI over empty vector-transfected cells. Data are represented as mean±s.e.m.;n=3, ***P(t-test)<0.0001. HeLa cells overexpressing GPx1 were stained with DCFDA-H2 and the change in fluorescence was observed by microscopy (i). Scale bar, 10 μm. Figure 5: Rescue of cell viability by Vn. ( a , b ) The viability of HEK293T cells under H 2 O 2 - or CuSO 4 -treated conditions along with other ROS modulators was observed through MTT assay and represented as mean±s.e.m. ; n =8, ** P ( t -test)<0.001. ( c , d ) Prevention of ROS-mediated apoptosis induction by nano-V 2 O 5 was analysed through the effector caspase-3/7 activity by measuring cleavage of specific substrate, resulting in the increase in fluorescence intensity. Bars denote the fold intensity over untreated cells as mean±s.e.m. ; n =3, *** P ( t -test) <0.0001. ( e , f ) The level of cellular GSH or GSSG was quantified in HEK293T cells treated with Vn and GSH inhibitor (BSO) using GSH/GSSG-Glo kit (Promega). Data are represented as mean±s.e.m. ; n =3, *** P ( t -test) <0.0001. ( g – i ) The GPx mimetic nature of Vn was confirmed by overexpressing GPx1 in HEK293T cells. Cells were transfected with pCDNA3.1a empty vector (EV) or vector containing GPx1. GPx1 overexpression was analysed in whole-cell lysate using the anti-GPx1 antibody ( g ). Anti-Flag tag antibody and anti-β-actin antibodies were used as transfection control and loading control, respectively. The cellular H 2 O 2 level was measured by staining the cells with Amplex Red after 48 h of transfection ( h ). Results are presented as fold change in MFI over empty vector-transfected cells. Data are represented as mean±s.e.m. ; n =3, *** P ( t -test)<0.0001. HeLa cells overexpressing GPx1 were stained with DCFDA-H2 and the change in fluorescence was observed by microscopy ( i ). Scale bar, 10 μm. Full size image In agreement with our previous ROS data, exposure of cells to the metal complex (Vc) resulted in higher cell death under both treated or untreated conditions. In contrast to Vn, the bulk material (Vb), the foam form (Vf) and the complexes (Vc, Vc 2 and Vc 3 ) lacked the ROS scavenging ability and had deleterious consequences for the cell viability ( Supplementary Fig. 7g,h ). Although Vb showed relatively lower antioxidant activity under in vitro conditions ( Supplementary Fig. 6a ), treatment of cells with Vb caused an intrinsic increase in the cellular free radical levels, which was further elevated on oxidative insult. Concurrently, the Vb-treated cells showed a sharp decrease in cell viability ( Supplementary Fig. 7g ). These data are in agreement with the EPR data that the metal ion in Vb undergoes reduction in the presence of GSH, which may lead to the generation of free radical species on reaction with H 2 O 2 ( vide infra and Supplementary Fig. 14b ). Lastly, we addressed the overall retention ability and toxicity of the Vn on longer time scale. We found that Vn did not have any detrimental effect on the cell viability and retained a significant degree of ROS scavenging activity even after 24 h post treatment ( Supplementary Figs 7e and 9b,c ). To rule out the possible involvement of cellular antioxidant machinery in Vn-mediated ROS scavenging through activation of oxidative stress-responsive transcription factors, we measured the expression level of downstream antioxidant enzymes in HEK293T cells. Analysis of the expression of Mn-superoxide dismutase (SOD-2), GPx1 and catalase in cells treated with Vn indicated no changes in the expression levels of these enzymes after Vn treatment. An increase in the expression of GPx1 after H 2 O 2 and 3-AT treatment was observed, which is probably due to the cellular defense mechanism in response to oxidative stress. The increase in GPx1 level was, however, restored in cells treated with Vn along with H 2 O 2 ( Supplementary Fig. 9d ). These results indicate that Vn itself acts as H 2 O 2 scavenger without involving cellular antioxidant machinery for the antioxidant effect. To test the effect of Vn on the redox signalling pathways in the cells, we analysed the expression of genes regulated by the major stress-responsive factor Nrf2 (ref. 43 ). The suppression of Nrf2 target genes’ expression was not observed when the cells were treated with Vn ( Supplementary Fig. 9e ), indicating that Vn does not interfere with the cellular redox sensing pathways, but it supplements the antioxidant system of the cell. Interestingly, although an upregulation of certain Nrf2 target genes such as glutamate–cysteine ligase catalytic (GCLC) and modifier (GCLM) subunits, and haem oxygenase-1 (HO-1) was observed under oxidative stress conditions (that is, in the presence of H 2 O 2 ), these protein expression levels were found to be normal in the presence of Vn ( Supplementary Fig. 9e ). This is presumably due to scavenging of H 2 O 2 by Vn that may prevent the stimulation of Nrf2 response. To further prove the intracellular GPx mimetic nature of Vn, we overexpressed the most abundant isoform of GPx, GPx1, in HEK293T cells and exposed the cells to H 2 O 2 treatment. We found through Amplex Red and DCFDA-H2 staining a decrease in total peroxide levels similar to that of Vn-pretreated cells, as analysed by flow cytometry and microscopy experiments ( Fig. 5g–i and Supplementary Fig. 19 ). The overexpression of GPx1 did not alter the expression pattern of different Nrf2 target genes. However, an upregulation of GCLC, GCLM and HO-1, observed after treatment with H 2 O 2 , was restored back to normal levels similar to Vn treatment ( Supplementary Fig. 9f ). In summary, our results prove that nano-V 2 O 5 (Vn) possess the unique property of scavenging intracellular ROS, prevents apoptotic trigger and protects cell viability by acting as a GPx enzyme mimetic by using GSH as a cofactor. The abundance of H 2 O 2 in the cell is more as compared with other ROS species and hence plays a critical role in cellular damage [44] . Therefore, cells have evolved a variety of peroxide metabolizing systems to maintain the ROS balance. However, under pathogenic conditions deregulated, ROS levels become the causative agent of pleiotropic defects giving rise to disease conditions. The robust ROS scavenging activity of Vn nanozyme even in the absence of catalase, one of the most potent H 2 O 2 degrading enzymes, underlines its applicability as an artificial enzyme to control ROS imbalance in the cells. Protection of ROS-induced damage of intracellular components The excess of free radicals generated in the cell mainly damage three major biomolecules, namely lipids, proteins and DNA [5] , [6] , [7] . Therefore, the cytoprotective role of Vn was analysed by measuring three parameters of intracellular damage such as lipid peroxidation, protein carbonylation and DNA strand breaks. The amount of lipid peroxides in the cell was quantified by measuring the levels of their decomposed highly reactive carbonyl product malondialdehyde [45] . We observed an increase in the amounts of lipid peroxides in the cells treated with Cu 2+ alone as compared with those pretreated with Vn ( Fig. 6f ). Similarly, cells left unexposed to Vn showed higher levels of protein carbonyls in comparison with Vn-containing cells in the presence or absence of Cu 2+ ( Fig. 6a,b and Supplementary Fig. 19 ). The level of protection against DNA damage by Vn was addressed by quantifying the number of phosphorylated γH 2 AX foci formed as a consequence of DNA double-strand breaks [5] . We found that Vn exerted a significant protective effect on DNA integrity and the cells accumulated lower amounts of intrastrand breaks than the nanowire-untreated cells ( Fig. 6e ). This is suggested by increased formation of γH 2 AX foci in the absence of Vn than in cells pretreated with nanowires, on oxidative insult. A similar effect was observed for calf thymus DNA in vitro in the presence of H 2 O 2 ( Supplementary Fig. 10 ). Depletion of intracellular GSH by AA or exposure of cells to Vc resulted in increased levels of lipid peroxides, protein carbonyls and γH 2 AX foci ( Fig. 6a,b,e,f ). As demonstrated above, in the latter case, redox reactions of Vc in cells cause these oxidative damages. These results underline that GSH is essential for the GPx-like activity of Vn nanozymes for their cytoprotective function. 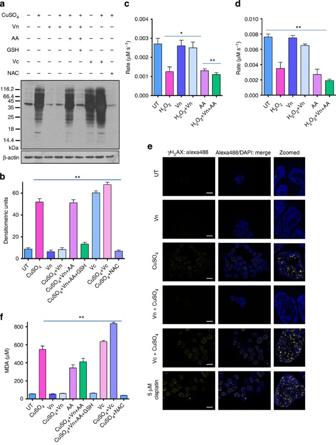Figure 6: Protection of cellular components from ROS-induced damage by Vn. (a,b) HEK293T cells subjected to treatment as indicated, were lysed and derivatized using 2,4-DNPH before SDS–PAGE and immunoblot analysis using anti-DNP antibodies.N-acetyl cysteine treated cells (NAC) (100 μM) were used as positive control. (b) The lanes were quantified and represented as fold densitometric values over untreated cells (c) The aconitase activity was quantified by recording an increase in absorbance at 240 nm for the production ofcis-aconitate. (d) Succinate dehydogenase activity was measured by coupling the reduction of ubiquinone to 2,6-dichlorophenolindophenol (DCPIP). The loss in blue colour due to reduction of DCPIP was monitored at 600 nm. (e) The amount of DNA double-strand break was analysed by detecting the foci formation by phosphorylated form of γH2AX through immunofluorescence microscopy. Data are represented as mean±s.e.m.;n=3, **P(t-test)<0.001, *P ((t-test)<0.01. Scale bar,10 μm. (f) The amount of lipid peroxidation was measured by quantifying the levels of malondialdehyde (MDA) in the cell lysate through thiobarbituric acid reactive substances assay. The extent of lipid peroxidation was represented as fold changes in absorbance recorded at 532 nm. Figure 6: Protection of cellular components from ROS-induced damage by Vn. ( a , b ) HEK293T cells subjected to treatment as indicated, were lysed and derivatized using 2,4-DNPH before SDS–PAGE and immunoblot analysis using anti-DNP antibodies. N -acetyl cysteine treated cells (NAC) (100 μM) were used as positive control. ( b ) The lanes were quantified and represented as fold densitometric values over untreated cells ( c ) The aconitase activity was quantified by recording an increase in absorbance at 240 nm for the production of cis -aconitate. ( d ) Succinate dehydogenase activity was measured by coupling the reduction of ubiquinone to 2,6-dichlorophenolindophenol (DCPIP). The loss in blue colour due to reduction of DCPIP was monitored at 600 nm. ( e ) The amount of DNA double-strand break was analysed by detecting the foci formation by phosphorylated form of γH 2 AX through immunofluorescence microscopy. Data are represented as mean±s.e.m. ; n =3, ** P ( t -test) < 0.001, * P ( ( t -test) < 0.01. Scale bar,10 μm. ( f ) The amount of lipid peroxidation was measured by quantifying the levels of malondialdehyde (MDA) in the cell lysate through thiobarbituric acid reactive substances assay. The extent of lipid peroxidation was represented as fold changes in absorbance recorded at 532 nm. Full size image It is known that mitochondria are the primary source of ROS via electron channelling through the respiratory complexes. An increase in the mitochondrial free-radical levels causes oxidation of the central Fe 2+ moiety of Fe–S cluster protein, resulting in loss of tetrahedral geometry and loss of enzyme function [46] , [47] . Therefore, we attempted to address the ability of Vn to protect the Fe–S cluster enzyme function from free-radical damage. These experiments were carried out by using two model Fe–S cluster enzymes, membrane-associated succinate dehydrogenase and matrix-localized aconitase. The activities of these enzymes under oxidative stress conditions in the presence of Vn were found to be comparable to that of controls ( Fig. 6c,d ), suggesting that Vn in the presence of GSH effectively protect the function of Fe–S cluster proteins and activities of the enzymes. Mechanistic details As mentioned earlier, the reaction follows enzyme-like mechanism as inferred from the Michaelis–Menten plots. The surface-exposed 010 planes ( Fig. 7a,b ) may act as catalytic sites, which are similar to the ones shown for the vanadium haloperoxidase activity of Vn [27] . To understand the interactions of GSH on the Vn surface, we carried out elemental X-ray mapping of sulfur and vanadium ( Supplementary Fig. 11a–c ), which indicates that GSH molecules are bound to the surface of Vn. Further, appearance of S2p signal in XPS of Vn-treated GSH confirms such interactions ( Supplementary Fig. 11d ). When the decrease in the concentration of NADPH was monitored at 340 nm, a complete reduction of H 2 O 2 was observed in the first cycle. However, subsequent addition of H 2 O 2 (240 μM) led to a further decrease in the NADPH concentration, indicating the stability and catalytic nature of Vn during the reduction ( Fig. 7c ). A similar profile was observed when the formation of GSSG was monitored by high-performance liquid chromatography (HPLC) ( Fig. 7d ). Treatment of Vn with H 2 O 2 alone led to the disappearance of a band at ~420 nm ( Fig. 7f ), which is probably due to the change in the functional groups on the surface by the formation of vanadium peroxido species 1 ( Fig. 8 ). Addition of an excess amount of GSH to 1 did not reproduce the band at 420 nm ( Fig. 7f ), indicating that the reaction follows a shunt pathway and regeneration of vanadium oxo is not necessary for the GPx-like activity ( Fig. 8 ). These observations were further supported by infrared analysis ( Supplementary Fig. 12a ). The ultraviolet–visible ( Fig. 7f ) and EPR ( Fig. 7g ) spectral analyses indicated that the oxidation state of vanadium in Vn was not affected by the addition of GSH. However, a partial reduction of vanadium(V) by H 2 O 2 leading to the formation of V(IV) and ·OOH was observed at liquid nitrogen temperature ( Supplementary Fig. 13a ) [31] . When the EPR was recorded at room temperature, the main unstructured signal almost disappeared, indicating a recombination of V(IV) and ·OOH to produce the peroxido species in which the vanadium is in the +5 oxidation state ( Fig. 7g ). The formation of peroxido species was also confirmed by Raman spectroscopic studies, which showed a sharp peak at 591 cm −1 with another peak at 1,200 cm −1 corresponding to the overtone [48] , [49] ( Supplementary Fig. 12b ). The small signal in the EPR spectrum of Vn+H 2 O 2 also suggests that the O–O bond in the peroxide complex is polarized. However, this small EPR signal disappeared completely after the treatment with an excess amount of GSH, suggesting that the GSH attacks on the polarized oxygen atoms of 1 ( Fig. 8 ). According to the mechanism ( Supplementary Fig. 13b ), the protonation (H + originating from GSH) and nucleophilic attack of GS − take place simultaneously at the oxygen atom that carries a partial negative charge ( δ -) and positive charge ( δ +), respectively. In contrast to Vn, the eight line patterns in EPR spectra suggest that the vanadium in Vc and Vb is reduced from +5 to +4 oxidation state on treatment with GSH ( Fig. 7g and Supplementary Fig. 14b ), which is probably responsible for the increase in the ROS level. The XPS data also confirm that the +5 oxidation state of vanadium centre in Vn is unaffected by GSH treatment ( Supplementary Fig. 14a ). Interestingly, the cyclic voltammograms show a significant difference in the redox potential of Vn as compared with that of Vb ( Supplementary Fig. 14c ) [50] , [51] . These observations confirm that the quantum size confinement of Vn alters the redox potential and enhances the stability of the +5 oxidation state of vanadium during the entire catalytic cycle. When a stronger reducing agent such as NaBH 4 is used, the vanadium centre does undergo a reduction as evidenced by a colour change from yellow (+5) to blue (+4) ( Supplementary Fig. 14d ). In the nanostructure, the surface of Vn acts as a template for the reduction of H 2 O 2 by GSH. The nucleophilic attack of GS − at the peroxide bond in complex 1 leads to the formation of an unstable sulfenate-bound intermediate 2 , which on hydrolysis generates glutathione sulfenic acid ( 3 , GSOH) and the dihydroxo intermediate 4 ( Fig. 8 ). The hydrolysis of 2 to produce GSOH is probably similar to the elimination of HOBr from V-OBr intermediate in vanadium haloperoxidase [27] . The formation of 3 was confirmed by HPLC and mass spectral analysis ( Supplementary Fig. 15a,b ). The reaction of 4 with H 2 O 2 regenerates the peroxido species 1 ( Fig. 8 ). This is similar to one of the steps proposed in the mechanism of vanadium chloroperoxidase [52] . The protonation of one of the hydroxyl units (HO − ) at vanadium centre by H 2 O 2 produces a water molecule and HOO − . The weakly bound water molecule then dissociates from the vanadium ion, which facilitates the attack of HOO − at vanadium, leading to the formation of a hydroperoxido species. A spontaneous elimination of another water molecule then generates the vanadium peroxido species ( Supplementary Fig. 16 ). The reaction of GSOH with GSH produces GSSG, which could be reduced to GSH by GR/NADPH. The formation of GSSG was also observed with Cum-OOH and t -BuOOH ( Fig. 7h ), although the antioxidant activity of Vn is more specific to H 2 O 2 . This is probably due to the formation of vanadium peroxido species, which were not produced when Vn was treated with Cum-OOH and t -BuOOH as seen from the Raman spectral data ( Supplementary Fig. 12b ). It should be noted that GSOH ( 3 ) undergoes further oxidation to produce the corresponding sulfinic acid ( 5 , GSO 2 H) at higher concentrations of H 2 O 2 ( Supplementary Fig. 17a,b ). In addition to GSH, other thiol-containing small molecules such as cysteine, cysteamine and mercaptoethanol can also be used as thiol cofactor. Vn exhibited significant thiol peroxidase activity by catalytically reducing H 2 O 2 in the presence of these thiols ( Supplementary Fig. 18 ). 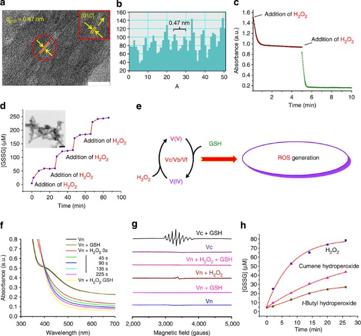Figure 7: Mechanistic investigation. (a) High-resolution TEM (HRTEM) images of the exposed plane 010 withd=0.47 nm, where the catalysis is known to take place. Inset is the magnified image of the highlighted part in HRTEM. Scale bar, 10 nm (b) The distance between the planes calculated by the software, Digital Micrograph. (c,d) The plots represent the mechanism is cyclic/catalytic. The activity was studied for two cycles in ultraviolet–visible spectroscopy by addition of H2O2(240 μM) and then following the decrease of NADPH at 340 nm. Similarly, GSSG was followed by HPLC for four cycles by the addition of H2O2(240 μM) at the end of each cycle. Inset shows the TEM image of the used Vn. Scale bar, 0.2 μm. (e) The redox recycling of vanadium in Vc and Vb. (f) Ultraviolet–visible spectra showing the band at ~420 nm (corresponding to the band gap of Vn) for Vn. The addition of GSH alone does not alter this band. However, the addition of H2O2leads to the disappearance of this band, which may indicate the formation of peroxido species on the surface of Vn. Reappearance of the band at ~420 nm was not observed after addition of excess GSH to the produced vanadium peroxido species. (g) EPR spectra shows that the vanadium in Vn does not undergo reduction after the addition of GSH. The appearance of a signal at 3,200 Gauss at liquid nitrogen temperature (Supplementary Fig. 13) due to (·OOH) almost disappeared at room temperature, indicating the recombination of ·OOH and V(IV) and the formation of peroxido species. Further, addition of GSH to the peroxido species does not result in the generation of V(IV), indicating the attack of thiolate (GS−) at the peroxido species. However, GSH reduces vanadium centre V(V) to V(IV) in Vc. (h) Selectivity studies between H2O2, Cum-OOH andt-BuOOH by HPLC analysis. The reaction of H2O2with Vn is much faster than that of Cum-OOH ort-BuOOH. Figure 7: Mechanistic investigation. ( a ) High-resolution TEM (HRTEM) images of the exposed plane 010 with d =0.47 nm, where the catalysis is known to take place. Inset is the magnified image of the highlighted part in HRTEM. Scale bar, 10 nm ( b ) The distance between the planes calculated by the software, Digital Micrograph. ( c , d ) The plots represent the mechanism is cyclic/catalytic. The activity was studied for two cycles in ultraviolet–visible spectroscopy by addition of H 2 O 2 (240 μM) and then following the decrease of NADPH at 340 nm. Similarly, GSSG was followed by HPLC for four cycles by the addition of H 2 O 2 (240 μM) at the end of each cycle. Inset shows the TEM image of the used Vn. Scale bar, 0.2 μm. ( e ) The redox recycling of vanadium in Vc and Vb. ( f ) Ultraviolet–visible spectra showing the band at ~420 nm (corresponding to the band gap of Vn) for Vn. The addition of GSH alone does not alter this band. However, the addition of H 2 O 2 leads to the disappearance of this band, which may indicate the formation of peroxido species on the surface of Vn. Reappearance of the band at ~420 nm was not observed after addition of excess GSH to the produced vanadium peroxido species. ( g ) EPR spectra shows that the vanadium in Vn does not undergo reduction after the addition of GSH. The appearance of a signal at 3,200 Gauss at liquid nitrogen temperature ( Supplementary Fig. 13 ) due to (·OOH) almost disappeared at room temperature, indicating the recombination of ·OOH and V(IV) and the formation of peroxido species. Further, addition of GSH to the peroxido species does not result in the generation of V(IV), indicating the attack of thiolate (GS − ) at the peroxido species. However, GSH reduces vanadium centre V(V) to V(IV) in Vc. ( h ) Selectivity studies between H 2 O 2 , Cum-OOH and t -BuOOH by HPLC analysis. The reaction of H 2 O 2 with Vn is much faster than that of Cum-OOH or t -BuOOH. 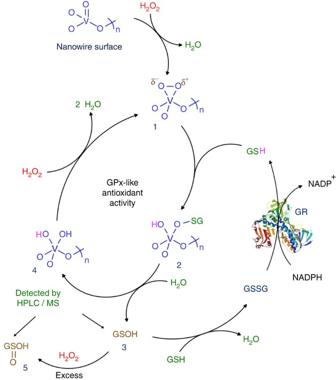Figure 8: Mechanism of GPx activity of Vn. Schematic diagram showing the molecular details of the mechanism of Vn nanozyme’s activity. The formation of peroxido species1was confirmed by Raman spectroscopic studies. Full size image Figure 8: Mechanism of GPx activity of Vn. Schematic diagram showing the molecular details of the mechanism of Vn nanozyme’s activity. The formation of peroxido species 1 was confirmed by Raman spectroscopic studies. Full size image In conclusion, this study suggests that Vn nanowires have the potential to be used as an antioxidant therapeutic agent for the host defense against ROS-mediated cellular damage under pathological conditions. ROS such as H 2 O 2 are generated as byproducts of the normal metabolism, but their levels are subdued due to a well-defined cellular antioxidant system. At the elevated ROS levels, the antioxidant defense mechanism fails to circumvent the detrimental effect of the free radicals, resulting in irreparable damage to biomolecules thereby causing severe oxidative stress. Organisms exposed to constant oxidative stress age quickly and are susceptible to multiple pathological conditions, including neurodegenerative diseases and neoplastic transformation. The deleterious effect of ROS-mediated cellular damages can be suppressed in several pathological conditions by synthetic compounds with potential antioxidant activity. Strikingly, the vanadia nanowires reported in this paper internalize in different cell types and display robust GPx mimetic activity under physiological conditions. The biocompatible Vn nanozyme exhibits significant cytoprotective effects against oxidative stress. Vn does not downregulate the endogenous antioxidant response, but rather, supplements the antioxidant system in mammalian cells. The Vn nanowires are able to completely suppress the ROS-mediated critical cellular damages such as protein oxidation, lipid peroxidation and DNA damages in the presence of glutathione, thus providing an important cytoprotection to the cell. Synthesis of Vn Vn were prepared by a hydrothermal method as described in the earlier report [27] . The mixture of VOSO 4 .H 2 O (8 mmol) and KBrO 3 (5 mmol) were stirred for 30 min in 30 ml of distilled water. The pH of the solution was adjusted to 2 by addition of nitric acid and transferred to a teflon-lined stainless steel autoclave. After the reaction period of 24 h at 180 °C, the autoclave was allowed to cool to room temperature and the precipitate was washed several times with water. As this material contains traces of V(IV) species, the precipitate was treated with small amount of t-butyl hydroperoxide. The resulting nanomaterial was washed several times with ultrapure water followed by ethanol and dried at 80 °C overnight under vacuum to get high-quality Vn. The Vn was well characterized by various methods. Absorption spectrum was acquired on Perkin-Elmer Lambda 35 ultraviolet–visible spectrophotometer. SEM images and EDX spectra were recorded on Fei Sirion UHR SEM and ESEM-Quanta instruments. TEM images, high-resolution TEM images and selected area electron diffraction pattern were recorded on JEOL 2100 instrument operating at 200 KV. Powder X-ray diffraction of Vn was obtained by PANalytical Xpert pro theta-two theta diffractometer using a CuKα (1.5406 Å) radiation. GPx-like activity of Vn The GPx-like catalytic activity of Vn was studied using the GR-coupled assay by following the decrease in the concentration of NADPH spectrophotometrically at 340 nm on a Perkin-Elmer Lambda 35 ultraviolet–visible spectrophotometer under time drive mode. In a typical assay (1 ml), the reactants were added in the following order, Vn (0.02 mg ml −1 ), GSH (2 mM), NADPH (0.4 mM), GR (1.7 units), H 2 O 2 (240 μM) in 100 mM, pH 7.4 phosphate buffer and reaction rate was followed for 30 s at 25 °C. The control reactions were performed in the absence of at least one of the reactants. The steady-state kinetics of Vn were studied by varying the concentration of Vn (0–0.02 mg ml −1 ), H 2 O 2 (0–480 μM) and GSH (0–6.0 mM) at a time and at the fixed concentration of GR and NADPH in 100 mM phosphate buffer (pH 7.4). Michaelis–Menten curves and Lineweaver–Burk plots were obtained by using origin 6.1 software. To understand the effect of haloperoxidase substrates on the GPx-like activity of Vn, the GPx-like activity of Vn was followed in the presence of KI (2 mM) and tyrosine or dopamine (2 mM) with GR-coupled assay in 100 mM phosphate buffer (pH 7.4). Cooperativity of Vn to work in a cascade To study the cooperativity of Vn with other enzymes, we employed GO in an assay to generate H 2 O 2 in situ using galactose as a substrate. Briefly, the GO (0.25 or 1 unit) was incubated with galactose (245 mM) for 1 min and then other reagents required for the GPx-like activity were added to the reaction mixture. The decrease in the concentration of NADPH was monitored at 340 nm by ultraviolet–visible spectrophotometry. Cell lines and cell culture HEK293T (Human Embryonic kidney cells ATCC Number: CRL-3216) and HeLa cells (ATCC Number: CCL-2) were grown in DMEM and Eagle’s minimum essential medium (Invitrogen), respectively, containing 10% fetal bovine serum (Gibco) and 1% penicillin–streptomycin (Gibco) at 37 °C in 5% CO 2 . LNCaP (ATCC Number: CRL-1740) and SH-SY5Y (ATCC Number: CRL-2266) cells were cultured in DMEM/F12 and RPMI 1640 (Invitrogen) medium, respectively, containing the above mentioned growth supplements. Cells were maintained at 60% confluency before measurement of ROS. Plasmids For the overexpression of GPx1, the ORF encoding GPx1 was amplified from HeLa cells complementary DNA library and cloned in pCDNA3.1a (+) vector under cytomegalovirus promoter. The GPx1 construct was transfected in HEK293T cells using Lipofectamine 2000 (Invitrogen). Empty pCDNA3.1a vector was transfected as a control for comparison. Measurement of ROS The cells were either left untreated or pretreated with 50 ng μl −1 of Vn (sonicated by probe sonicator for 5 min) before oxidative insult. The cellular monolayer was washed thoroughly by 1 × phosphate-buffered saline to remove the unincorporated nanoparticles. Oxidative stress was induced by exposing the cells to 200 μM H 2 O 2 , 500 μM CuSO 4 or 20 mM 3-amino-1,2,4-triazole for 15 min at 37 °C. AA (0.1 mM) and 50 μM BSO were used (for 15 min) to deplete the cellular GSH levels [38] . Replenishment of GSH was done by extensively washing the cells with 1 × phosphate-buffered saline to remove the AA or BSO, followed by addition of 100 μM GSH for 5 min. The effect of vanadium complexes was assessed by exposing the cells to 50 ng μl −1 of complexes for 15 min. After treatment, cells were trypsinized, washed with 1 × phosphate-buffered saline and stained with 15 μM DCFDA-H2 for 10 min at 30 °C. Ten thousand events were analysed by flow cytometry and the respective mean fluorescence intensity values were co-related with the ROS levels. For fluorescence microscopy, 5,000 cells were seeded and treated with ROS-modulating agents as stated above. Post treatment, the cells were stained with 5 μM DCFDA-H2. Images were acquired by Zeiss AxioObserver Z1 Apotome 2.0 63 x numerical aperture 1.45, Zeiss AxioCam MRm camera at a constant exposure of 300 ms and processed using Zeiss Axiovision Rel.4.8 software. For measurement of ROS using HyPer probe, the cells were transfected with the plasmid encoding HyPer (Evrogen) using Lipofectamine 2000 (Invitrogen). Post 48 h incubation, the cells were similarly treated as mentioned above and the relative HyPer fluorescence intensity was analysed using Tecan infinite Pro-200 spectrofluorometer. Amplex Red (Molecular Probes; Invitrogen) staining was performed following the manufacturer’s instructions. Cell viability and apoptosis The relative viability of cells was determined by MTT assay kit (Invitrogen) according to manufacturer’s instructions. The induction of apoptosis was measured by analysing caspase 3/7 activity as per the manufacturer’s protocol supplied in caspase-activity detection kit (Promega). The treatment of the cells was carried out similar to the protocol followed for ROS measurement. Measurement of cellular GSH and GSSG levels To measure the cellular level of GSH and GSSG, HEK293T cells were treated with Vn, H 2 O 2 and BSO as mentioned previously, followed by GSH/GSSG quantification using GSH/GSSH-Glo kit (Promega) as per the manufacturer’s instructions. Internalization of Vn in mammalian cells Approximately 20,000 HEK293T cells were seeded and allowed to grow overnight. The cells were treated with the vanadium nanowires for 15 min and then subjected to 3% paraformaldehyde fixation for 2 h. The fixed cells were dehydrated through alcohol gradient and allowed to air dry at room temperature. Further, the dried cells were sputtered with gold and images were recorded by SEM. The vanadium content was analysed by EDX spectroscopy. For the flow cytometry analysis, 1 × 10 5 HEK293T cells were treated with increasing concentrations (10, 25, 50, 100 and 150 ngμl −1 ) of Vn for 15 min. The cells were harvested by trypsinization and the change in the side scatter due to uptake of nanowires was analysed by flow cytometry [34] , [35] . As a control, equivalent concentrations of a soluble vanadium complex were used. For the quantification, ~60 million HEK293T cells were exposed to Vn, followed by cell lysis and ionization by addition of the concentrated nitric acid for 20 h. The samples were analysed by ICP-AES. Protein carbonylation Approximately 12 million cells were treated essentially as mentioned for the detection of ROS. Post treatment, the cells were harvested and lysed in RIPA buffer (50 mM Tris-HCl pH 7.6, 150 mM NaCl, 1% deoxycholate, 0.1% SDS, 1 mM phenylmethylsulfonyl fluoride). Equivalent amount of proteins was analysed for carbonylation through OxyBlot Protein Oxidation Detection Kit (Millipore), following the manufacturer’s instructions. Lipid peroxidation Treated or untreated HEK293T cells were harvested and sonicated at 30% amplitude for 3 pulses of 20 s. The cell lysate was incubated with 1% thiobarbituric acid for 1 h at 90 °C. The samples were centrifuged at 16,000 g for 3 min and the colour developed in the supernatant fraction was quantified spectrophotometrically at 530 nm. Assessment of DNA damage Approximately 20,000 cells were incubated with Vn for 15 min. Cells were fixed with 3% formaldehyde followed by a treatment with 90% methanol. The samples were washed with 1 × phosphate-buffered saline and blocked with 0.05% IgG-free BSA with 0.05% TritonX-100 for 30 min. After washing two times with 1 × phosphate-buffered saline, cells were incubated with anti- γH 2 AX antibody for 1 h. Secondary antibody detection was performed by Alexa488-conjugated antibody. Images were acquired using Zeiss AxioObserver Z1 Apotome 2.0 63 × numerical aperture 1.45. Images were digitally zoomed by Adobe Photoshop 7.0. Measurement of Fe–S cluster enzyme activity Measurement of Fe–S cluster enzyme activity was performed as described [53] , [54] . Briefly, succinate dehydrogenase activity was measured after activation of the complex by incubation with 20 mM succinate for 10 min at 30 °C. After the inhibition of other three respiratory complexes, 65 μM ubiquinone was added as an electron acceptor. The reduction of ubiquinone was coupled to formation of reduced 2,6-dichlorophenolindophenol. The loss in blue colour of 2,6-dichlorophenolindophenol was measured at 600 nm. Aconitase activity was carried out according to the procedure described [53] . Electron paramagnetic spectroscopy The formation of vanadium peroxido species and change in oxidation states were performed on Bruker ER 041X Microwave Bridge X-band EPR spectrometer. The spectrum was recorded by addition of H 2 O 2 (7%, 30 μl) to the capillary tube containing Vn (4 mg), followed by quenching in liquid N 2 and at room temperature. Control experiments were carried out in the same condition, with addition of GSH (25 mM, 30 μl) to Vn alone and vanadium peroxido species formed on Vn. Similarly, Vc (4 mg) and bulk V 2 O 5 (4 mg) in the presence of GSH was also analysed. HPLC analysis of GSH to GSSG conversion The reaction mixture was produced in such a way that it contained 0.02 mg Vn, 2 mM GSH, 240 μM H 2 O 2 in 1 ml H 2 O. This mixture was incubated in the auto sampler and injected automatically using 10 μl each at the appropriate time. The formation of GSSG was followed at 220 nm using Waters 2695 HPLC instrument having automatic injection system equipped with photodiode array detector. Intermediates such as GSOH and GSO 2 H were also detected by HPLC analysis and confirmed by mass spectroscopy using Bruker esquire 6000 mass spectrometer working in electron spray ionization mode. Antibodies and immunoblotting Immunodetection of catalase, GPx1 and SOD2 was performed using the antibodies, anti-catalase (Calbiochem, 1:4,000), anti-GPx1 (Pierce Thermo Scientific, 1:2,000) and anti-SOD2 (Pierce Thermo Scientific, 1:500), respectively. The other specific antibodies, anti-Prx3 (Pierce Thermo Scientific, 1:5,000), anti-FTH1 (Pierce Thermo Scientific, 1:500), anti-FLT1 (Pierce Thermo Scientific, 1:1,000), anti-TrxR1 (Pierce Thermo Scientific, 1:1,000), anti-Trx (Pierce Thermo Scientific, 1:1,000), anti-GCLM (Pierce Thermo Scientific, 1:1,000), anti-GCLC (Pierce Thermo Scientific, 1:500) and anti-HO-1 (Pierce Thermo Scientific, 1:500) were used to detect the expression profile of respective proteins. Anti-β-actin (Sigma, 1:20,000) was used as a loading control. The secondary detection was performed using horseradish peroxidase-conjugated anti-rabbit IgG (GE Amersham 1:20,000) or anti-mouse IgG (GE Amersham 1:10,000), and visualized by ECL chemiluminescent reagent (GE Amersham). Electrode preparation and cyclic voltammetric analysis For electrochemical studies, Vn and Vb electrodes were fabricated on stainless steel (SS) disks as the current collectors. Briefly, a commercial-grade SS foil disk (diameter 16 mm) was dipped in 30% dilute HNO 3 for about 5 min, washed several times with ultrapure water followed by acetone and dried in air. A mixture of Vn/Vb (90 wt %), acetylene carbon black (Alfa Aesar) (5 wt %) and polyvinylidene difluoride (5 wt %) was ground and a few drops of N -Methyl-2-pyrrolidone were added to get an ink, which was applied on the pre-treated SS disk of area 2.0 cm 2 . The disk was dried at 100 °C for about 30 min. The coating and drying steps were repeated to achieve a loading level of 6.0 mg cm −2 . Finally, the electrodes were dried at 110 °C under vacuum for 12 h. Coin-type cells (CR 2025) were assembled using a Li foil for the counter electrode in coin cell containers purchased from Hohsen Corporation, Japan. Before the cell assembly, the surface of Li ribbon was scraped to remove surface film. A microporous polypropylene film (Celgard model 2400) was used as the separator and the electrolyte was 1 M LiPF 6 in 1:1 (v/v) mixed solvents of dry ethylene carbonate and dimethyl carbonate. All the manipulations such as preparation of the mixed solvent, its purification, electrolyte preparation and cell assembly were carried out in an Ar atmosphere using a glove box (MBraun model UNILAB). The cyclic voltammetry was performed in a potential range from 2.00 to 4.00 V at 0.1 mV s −1 scan rate. How to cite this article: Vernekar, A. A. et al. An antioxidant nanozyme that uncovers the cytoprotective potential of vanadia nanowires. Nat. Commun. 5:5301 doi: 10.1038/ncomms6301 (2014).